Integration of carbohydrate metabolism and redox state controls dauer larva formation inCaenorhabditis elegans Under adverse conditions, Caenorhabditis elegans enters a diapause stage called the dauer larva. External cues signal the nuclear hormone receptor DAF-12, the activity of which is regulated by its ligands: dafachronic acids (DAs). DAs are synthesized from cholesterol, with the last synthesis step requiring NADPH, and their absence stimulates dauer formation. Here we show that NADPH levels determine dauer formation in a regulatory mechanism involving key carbohydrate and redox metabolic enzymes. Elevated trehalose biosynthesis diverts glucose-6-phosphate from the pentose phosphate pathway, which is the major source of cellular NADPH. This enhances dauer formation due to the decrease in the DA level. Moreover, DAF-12, in cooperation with DAF-16/FoxO, induces negative feedback of DA synthesis via activation of the trehalose-producing enzymes TPS-1/2 and inhibition of the NADPH-producing enzyme IDH-1. Thus, the dauer developmental decision is controlled by integration of the metabolic flux of carbohydrates and cellular redox potential. When overcrowded or starved, Caenorhabditis elegans interrupts its reproductive cycle to enter diapause by forming a dauer (enduring) larva [1] . Dauer larvae can withstand extreme conditions such as treatment with strong detergents and severe desiccation [2] , [3] . This increased stress resistance is due to the reprogramming of gene expression that is radically different from that of reproductive larvae [4] , [5] . Similar gene expression changes are also found in long-living mutants [6] . Dauer larvae are broadly used as a paradigm for studying hypometabolism and metabolism during starvation [7] . Thus, understanding the mechanisms of dauer formation can shed light on general processes, such as ageing and decreased metabolic activity. Biochemical and genetic studies show that dauer formation is initiated by specific short-chain ascarosides acting as dauer-inducing pheromones [8] , [9] and is controlled by the so-called daf genes (for abnormal da uer f ormation). Three signalling pathways, namely the transforming growth factor (TGF)-β-like (defined by the TGF-β homologue DAF-7), insulin-like (defined by the insulin receptor homologue DAF-2) and cyclic GMP pathways [1] , converge on the activity of a nuclear hormone receptor/transcription factor, DAF-12 (refs 10 , 11 ). DAF-12 binds sterol-derived, bile acid-like molecules known as dafachronic acids (DAs) [12] , [13] . The last, crucial reaction in DA biosynthesis is catalysed by cytochrome P450 (CYP450) DAF-9, which produces a carboxyl group at the C-26 methyl residue of the precursor in three oxidation steps. This reaction requires NADPH [13] . DAF-9 is expressed in a pair of DA-secreting neuroendocrine cells called the XXX cells [14] . DAF-9 expression is also observed in the hypodermis, which is the syncytial epidermal tissue that surrounds the worm [14] . Secreted DAs act to suppress dauer-promoting activity of DAF-12 at the organism-wide level, and worms remain in the reproductive cycle [13] . Downregulation of DAF-7 or DAF-2 presumably reduces the level of available DA by inhibiting its synthesis, degrading it or sequestering it in an inactive form. One of the mechanisms regulating biosynthesis of DA may be the modulation of the concentration of substrates required for its synthesis. Recently, we showed that methylation of cholesterol in the fourth position by the sterol methylase STRM-1 renders cholesterol unsuitable for DA synthesis [15] . Another cofactor for DA production is cytosolic NADPH, which is used by DAF-9 as an electron donor [13] . Before this study, no information regarding the involvement of NADPH in the regulation of DA synthesis was available. Here we show that the level of cytosolic NADPH determines dauer formation and is regulated by the biosynthesis of the disaccharide trehalose, which diverts glucose-6-phosphate (G6P) from the pentose phosphate pathway (PPP), the major source of NADPH in the cell. We also show that DAF-12 negatively regulates DA production by two parallel mechanisms. First, DAF-12 increases the biosynthesis of trehalose by activating the enzymes TPS-1 and TPS-2. Second, DAF-12 downregulates IDH-1, another enzyme involved in NADPH production in the cytosol. Thus, the developmental switch (reproductive to dauer) is directly connected to the metabolic flux of carbohydrates as well as to cellular redox potential. Trehalose-deficient mutants exhibit reduced dauer formation Recently, we showed that dauer larvae produce stage-specific glycolipids (maradolipids) containing the disaccharide trehalose [16] . Here we exploited a C. elegans strain that was unable to synthesize trehalose to investigate whether trehalose production could also be involved in the determination of dauer fate. C. elegans produces trehalose from G6P and UDP-glucose in a two-step reaction [17] , [18] . In the first step, trehalose-6-phosphate is synthesized by trehalose-6-phosphate synthase (TPS), which is encoded by the genes tps-1 and tps-2 . Next, the phosphate is removed by trehalose-6-phosphate phosphatase. We produced a mutant C. elegans strain that lacked functional TPS-1 and TPS-2 proteins (ΔΔ tps ) and consequently was unable to synthesize trehalose [16] . We noticed that ΔΔ tps had a reduced number of dauers when grown in a liquid culture at high population density. The ΔΔ tps dauers, however, had proper dauer morphology as examined using electron microscopy [16] and were resistant to SDS treatment. To investigate the dauer formation in ΔΔ tps under controlled conditions, we tested dauer formation in the presence of synthetic dauer-inducing pheromones. As seen in Fig. 1a , ΔΔ tps formed approximately sevenfold fewer dauers than wild-type worms. This suggests that biosynthesis of trehalose is involved in the regulation of dauer formation. 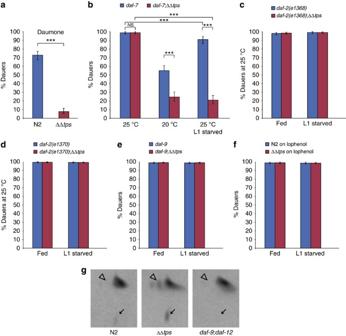Figure 1: Loss of TPS activity suppresses dauer formation by elevation of DA levels. (a) ΔΔtps(n=1,070) has diminished sensitivity to dauer pheromones in comparison with the wild type (N2,n=1,277). (b) Dauer formation ofdaf-7anddaf-7;ΔΔtps. ΔΔtpscauses a decrease in the Daf-c phenotype ofdaf-7at the semipermissive temperature (20 °C) and, when starved in L1 larva, at the restrictive temperature (25 °C). Fordaf-7: 25 °Cn=808, 20 °Cn=755, 25 °C L1 starvedn=855. Fordaf-7;ΔΔtps: 25 °Cn=906, 20 °Cn=744, 25 °C L1 starvedn=697. (c) Dauer formation ofdaf-2(e1368)anddaf-2(e1368);ΔΔtpsat restrictive temperature with or without starvation in L1. ΔΔtpsdoes not change the dauer formation ofdaf-2(e1368). Fordaf-2(e1368): fedn=627, L1 starvedn=566. Fordaf-2(e1368);ΔΔtps: fedn=705, L1 starvedn=650. (d) Dauer formation ofdaf-2(e1370)anddaf-2(e1370);ΔΔtpsat restrictive temperature. Starvation in L1 was also examined. ΔΔtpsdoes not change the dauer formation ofdaf-2(e1370). Fordaf-2(e1370): fedn=618, L1 starvedn=660. Fordaf-2(e1370);ΔΔtps: fedn=452, L1 starvedn=446. (e) Dauer formation ofdaf-9anddaf-9;ΔΔtpswith or without starvation in L1. ΔΔtpsdoes not change the formation of dauer larvae ofdaf-9. Fordaf-9: fedn=231, L1 starvedn=231. Fordaf-9;ΔΔtps: fedn=204, L1 starvedn=220. (f) Dauer formation observed on medium in which cholesterol is replaced by lophenol with or without starvation in L1. ΔΔtpsis not sufficient for a substantial decrease in dauer larvae. For N2: fedn=512, L1 starvedn=533. For ΔΔtps: fedn=445, L1 starvedn=412. (g) Detection of DA (arrowheads) and the putative (25S)-3α-hydroxy-7-cholestanoic acid (arrows) by 2D-TLC of extracts of3H-cholesterol labelled worms. ΔΔtpshas increased intensity of the DA and cholestanoic acid bands in comparison with the wild-type (N2).daf-9;daf-12is unable to produce DA and cholestanoic acid because it lacks DAF-9. Scans of whole TLC plates are shown inSupplementary Fig. 1. In (a–f), data were collected from at least four biological replicates, from at least two experiments. Ing, representative images from two experiments. Error bars represent 95% confidence intervals. Means, confidence intervals and statistical significance were modelled by beta regression analysis. ***P<0.001; ns, no significant difference (beta regression). Figure 1: Loss of TPS activity suppresses dauer formation by elevation of DA levels. ( a ) ΔΔ tps ( n =1,070) has diminished sensitivity to dauer pheromones in comparison with the wild type (N2, n =1,277). ( b ) Dauer formation of daf-7 and daf-7; ΔΔ tps . ΔΔ tps causes a decrease in the Daf-c phenotype of daf-7 at the semipermissive temperature (20 °C) and, when starved in L1 larva, at the restrictive temperature (25 °C). For daf-7 : 25 °C n =808, 20 °C n =755, 25 °C L1 starved n =855. For daf-7; ΔΔ tps : 25 °C n =906, 20 °C n =744, 25 °C L1 starved n =697. ( c ) Dauer formation of daf-2(e1368) and daf-2(e1368); ΔΔ tps at restrictive temperature with or without starvation in L1. ΔΔ tps does not change the dauer formation of daf-2(e1368) . For daf-2(e1368) : fed n =627, L1 starved n =566. For daf-2(e1368); ΔΔ tps : fed n =705, L1 starved n =650. ( d ) Dauer formation of daf-2(e1370) and daf-2(e1370); ΔΔ tps at restrictive temperature. Starvation in L1 was also examined. ΔΔ tps does not change the dauer formation of daf-2(e1370) . For daf-2(e1370) : fed n =618, L1 starved n =660. For daf-2(e1370); ΔΔ tps : fed n =452, L1 starved n =446. ( e ) Dauer formation of daf-9 and daf-9; ΔΔ tps with or without starvation in L1. ΔΔ tps does not change the formation of dauer larvae of daf-9 . For daf-9 : fed n =231, L1 starved n =231. For daf-9; ΔΔ tps : fed n =204, L1 starved n =220. ( f ) Dauer formation observed on medium in which cholesterol is replaced by lophenol with or without starvation in L1. ΔΔ tps is not sufficient for a substantial decrease in dauer larvae. For N2: fed n =512, L1 starved n =533. For ΔΔ tps : fed n =445, L1 starved n =412. ( g ) Detection of DA (arrowheads) and the putative (25 S )-3α-hydroxy-7-cholestanoic acid (arrows) by 2D-TLC of extracts of 3 H-cholesterol labelled worms. ΔΔ tps has increased intensity of the DA and cholestanoic acid bands in comparison with the wild-type (N2). daf-9;daf-12 is unable to produce DA and cholestanoic acid because it lacks DAF-9. Scans of whole TLC plates are shown in Supplementary Fig. 1 . In ( a – f ), data were collected from at least four biological replicates, from at least two experiments. In g , representative images from two experiments. Error bars represent 95% confidence intervals. Means, confidence intervals and statistical significance were modelled by beta regression analysis. *** P <0.001; ns, no significant difference (beta regression). Full size image Next, we investigated the connection between the biosynthesis of trehalose and the major dauer-regulatory pathways. The TGF-β ( daf-7 ) pathway acts downstream of dauer-inducing pheromones [19] , [20] . A C. elegans strain bearing the daf-7 (e1372) allele has a dauer-constitutive (Daf-c) phenotype and forms ∼ 100% dauers at 25 °C (restrictive temperature) and ∼ 50% dauers at 20 °C (semipermissive temperature) [21] . To investigate whether tps-1 and tps-2 genetically interact with daf-7 , we introduced ΔΔ tps to a daf-7 background. As seen in Fig. 1b , the deficiency in trehalose biosynthesis significantly reduced the Daf-c phenotype of daf-7 at the semipermissive temperature (20 °C). Moreover, ΔΔ tps decreased dauer formation of daf-7 even at 25 °C when the L1 larvae were starved for 48 h before being transferred to the restrictive temperature ( Fig. 1b ). This effect was probably caused by the increase in DAF-9 expression on starvation, as described previously [22] . Thus, ΔΔ tps leads to a conditional, dauer-defective (Daf-d) phenotype and genetically interacts with the daf-7 pathway. In parallel to DAF-7, dauer formation is controlled by the insulin receptor-like protein DAF-2 (ref. 23 ). Mutation of this protein leads to a Daf-c phenotype [24] . Two distinct classes of daf-2 Daf-c alleles exist that are classified according to the ability of daf-12 Daf-d mutations to suppress the Daf-c phenotype and restore the reproductive development. Class I alleles (for example, daf-2(e1368) ) are rescued; however, class II alleles (for example, daf-2(e1370) ) are not rescued by daf-12 mutations [24] . To test the genetic interaction of tps-1/tps-2 with daf-2 , ΔΔ tps was placed in the background of the thermosensitive Daf-c mutations daf-2(e1368) and daf-2(e1370) . In contrast to the daf-7 pathway, ΔΔ tps could not suppress the Daf-c phenotypes of the class I or class II alleles of daf-2 under any of the conditions tested, including starvation in L1 ( Fig. 1c,d ). This suggests that a decrease in insulin signalling can induce dauer formation even when trehalose cannot be produced. The fact that biosynthesis of trehalose can influence dauer formation prompts the question as to whether this process acts upstream or downstream of the DA-producing enzyme DAF-9. To address this, we first investigated whether ΔΔ tps could suppress the Daf-c phenotype of daf-9 . Mutants bearing the null allele daf-9(dh6) produce dauer-like larvae because DA is not synthesized [13] , [14] , [22] . In the absence of exogenous DA, the triple mutant daf-9 ;ΔΔ tps could not produce reproductive adults under any of the conditions tested (with or without starvation; Fig. 1e ). Second, ΔΔ tps could not suppress the induction of wild-type dauers on substitution of cholesterol by lophenol. As previously shown, DA cannot be produced when lophenol is the only dietary sterol because cholesterol, the precursor for DA synthesis, is absent [25] . ΔΔ tps formed dauer larvae on lophenol and this process was not decreased by starvation ( Fig. 1f ). Since the absence of trehalose does not suppress either the null mutant of daf-9 or the absence of substrate for DA synthesis, it can be surmised that trehalose acts upstream or at the level of DAF-9. In the light of these findings, we expected that the absence of trehalose synthesis would increase the amount of DA. This hypothesis was tested by labelling worms with radioactive cholesterol and analysing the lipid extracts by two-dimensional (2D) thin-layer chromatography (2D-TLC). As seen in Fig. 1g and Supplementary Fig. 1 , ΔΔ tps produced substantially more DA than the wild type. A compound probably corresponding to (25 S )-3α-hydroxy-7-cholestanoic acid, a reduced form of DA that has also been proposed as an endogenous ligand of DAF-12 (refs 12 , 15 , 26 ) was also elevated in ΔΔ tps ( Fig. 1g ). Overexpression of TPS-1 enhances dauer formation Deficiency of trehalose biosynthesis resulted in decreased dauer formation. We therefore reasoned that overproduction of trehalose might have the opposite effect. A transgenic approach was employed to overexpress TPS [27] . We chose to overexpress one of the TPS enzymes, TPS-1. TPS-1 and TPS-2 have largely overlapping expression patterns and share high sequence similarity (54% identity, 71% similarity, WormBase WS246). A worm expression vector was constructed that contained eGFP (enhanced green fluorescent protein)-tagged tps-1 downstream of the putative endogenous tps-1 promoter ( Fig. 2a ). Transformed worm strains bearing an extrachromosomal array were selected as these presumably held multiple copies of the construct. 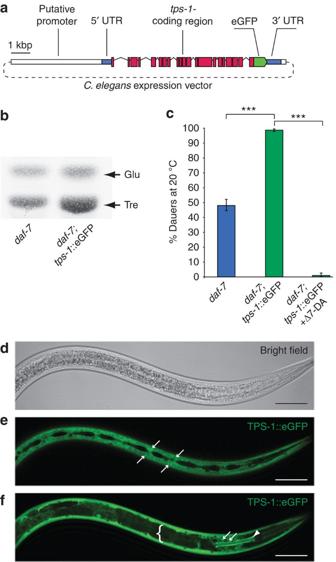Figure 2: Overexpression of TPS-1 leads to elevation of trehalose levels and dauer formation. (a) Design of the modified fosmid construct used for overexpression of TPS-1 indaf-7. The construct contains thetps-1-coding sequence tagged with eGFP at the C terminus with the corresponding endogenous 5′-untranslated region (UTR), 3′-UTR and∼5 kb promoter region. (b) TLC of sugars fromdaf-7anddaf-7;tps-1::eGFP. Sugars were visualized with Molisch reagent (Tre—trehaloseRf∼0.46, Glu—glucoseRf∼0.57). A scan of the whole TLC plate is shown inSupplementary Fig. 2. (c) Dauer formation ofdaf-7anddaf-7;tps-1::eGFP at 20 °C. Overexpression of TPS-1 enhances the Daf-c phenotype ofdaf-7, but the dauer formation is abolished in DA-fed animals.daf-7 n=746,daf-7;tps-1::eGFPn=756,daf-7;tps-1::eGFP+DAn=660. (d) Transmitted light micrograph of adaf-7;tps-1::eGFP animal grown at 20 °C. (e) Confocal scanning micrograph of the animal ind. TPS-1::eGFP fluorescence is detected in hypodermal syncytium (arrows). (f) In addition, TPS-1::eGFP is located to the isthmus of the pharynx (arrowhead) and the cell bodies of various head neurons (arrows). Intestinal cells are completely devoid of TPS-1::eGFP signal (curly bracket). Scale bars ind–f, 20 μm. Inb,d,e,f, representative images from at least two experiments. Inc, data were collected from six biological replicates from three independent experiments. Error bars represent 95% confidence intervals. Means, confidence intervals and statistical significance were modelled by beta regression analysis. ***P<0.001 (beta regression). Figure 2: Overexpression of TPS-1 leads to elevation of trehalose levels and dauer formation. ( a ) Design of the modified fosmid construct used for overexpression of TPS-1 in daf-7 . The construct contains the tps-1- coding sequence tagged with eGFP at the C terminus with the corresponding endogenous 5′-untranslated region (UTR), 3′-UTR and ∼ 5 kb promoter region. ( b ) TLC of sugars from daf-7 and daf-7;tps-1 ::eGFP. Sugars were visualized with Molisch reagent (Tre—trehalose R f ∼ 0.46, Glu—glucose R f ∼ 0.57). A scan of the whole TLC plate is shown in Supplementary Fig. 2 . ( c ) Dauer formation of daf-7 and daf-7;tps-1 ::eGFP at 20 °C. Overexpression of TPS-1 enhances the Daf-c phenotype of daf-7 , but the dauer formation is abolished in DA-fed animals. daf-7 n =746, daf-7;tps-1 ::eGFP n =756, daf-7;tps-1 ::eGFP+DA n =660. ( d ) Transmitted light micrograph of a daf-7;tps-1 ::eGFP animal grown at 20 °C. ( e ) Confocal scanning micrograph of the animal in d . TPS-1::eGFP fluorescence is detected in hypodermal syncytium (arrows). ( f ) In addition, TPS-1::eGFP is located to the isthmus of the pharynx (arrowhead) and the cell bodies of various head neurons (arrows). Intestinal cells are completely devoid of TPS-1::eGFP signal (curly bracket). Scale bars in d – f , 20 μm. In b , d , e , f , representative images from at least two experiments. In c , data were collected from six biological replicates from three independent experiments. Error bars represent 95% confidence intervals. Means, confidence intervals and statistical significance were modelled by beta regression analysis. *** P <0.001 (beta regression). Full size image Under normal growth conditions, the overexpression of tps-1 did not produce a Daf-c phenotype. To test dauer formation under mild dauer-inducing conditions, the tps-1 -overexpressing strain was crossed to daf-7 to obtain daf-7;tps-1::eGFP . Biochemical analysis showed that daf-7;tps-1::eGFP produced more trehalose than daf-7 ( Fig. 2b and Supplementary Fig. 2 ). This transgenic line was strongly Daf-c: at 20 °C, ∼ 100% dauers were formed ( Fig. 2c ). The effect of tps-1::eGFP on dauer formation was, however, fully abolished when DA was added to the medium, again demonstrating that biosynthesis of trehalose stimulated dauer formation by interfering with DA synthesis ( Fig. 2c ). Light microscopy was performed on daf-7;tps-1 ::eGFP undergoing dauer formation to investigate the localization of TPS-1 ( Fig. 2d–f ). Strong expression occurred predominantly in the hypodermis ( Fig. 2e ), a tissue in which DAF-9 and STRM-1 are also expressed [14] , [15] , [22] . Some expression was observed in a number of head neurons and in the isthmus of the pharynx, and no expression was seen in the intestinal cells ( Fig. 2f ). Thus, overexpression of TPS-1 might enhance dauer formation by acting in the cells responsible for DA synthesis (hypodermis). Availability of cytosolic NADPH determines dauer formation We next wished to investigate how the absence of trehalose might lead to a reduction in dauer formation. One possible explanation is that trehalose is itself a dauer-inducing molecule. However, feeding daf-7 with even very high amounts of trehalose had no effect on dauer formation ( Fig. 3a ). Therefore, we hypothesized that the biosynthesis of trehalose and DA is coupled. 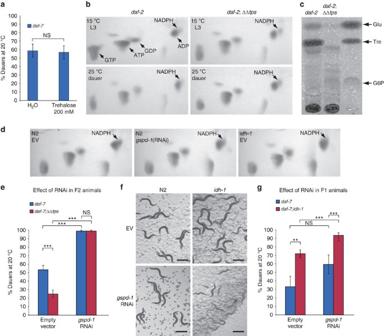Figure 3: Cellular NADPH levels determine dauer formation. (a) High concentration of trehalose in the feeding medium does not enhance the Daf-c phenotype ofdaf-7. Control (water)n=684, trehalose treatedn=612. (b) 2D-TLC of nucleotides fromdaf-2(e1370)anddaf-2(e1370);ΔΔtpsL3 and dauer larvae. ΔΔtpscauses marked increase in NADPH in both L3 and dauer larvae ofdaf-2. (c) TLC of sugars fromdaf-2(e1370)anddaf-2(e1370);ΔΔtpsdauers. Note the disappearance of the trehalose band and the accumulation of G6P indaf-2;ΔΔtps(G6P—glucose-6-phosphateRf∼0.17, Tre—trehaloseRf∼0.46, Glu—glucoseRf∼0.57). (d) 2D-TLC of nucleotides derived from wild-type (N2) L3 larvae after two generations on empty vector control RNAi (EV) orgspd-1(RNAi) andidh-1(ok2832)on EV. Note the reduction of the NADPH levels caused bygspd-1(RNAi). The mutant ofidh-1also displays lower NADPH amounts compared with the wild type. Scans of whole TLC plates are shown inSupplementary Figs 3–5. (e) Dauer formation ofdaf-7anddaf-7;ΔΔtpsongspd-1(RNAi) at 20 °C.gspd-1(RNAi) leads to an increase in the incidence of dauers. Fordaf-7: EVn=775,gspd-1(RNAi)n=782. Fordaf-7;ΔΔtps: empty vectorn=814,gspd-1(RNAi)n=734. (f) When PPP is partially inactivated by RNAi againstgspd-1, in the first generation the wild-type worms do not have obvious defects. Under the same conditions,idh-1mutants display pronounced slow growth, sick and reduced body size phenotypes. Scale bars, 500 μm. (g) Dauer formation ofdaf-7anddaf-7;idh-1ongspd-1(RNAi) at 20 °C.daf-7;idh-1shows higher incidence of dauers compared withdaf-7and it is further enhanced bygspd-1(RNAi). Fordaf-7: empty vectorn=823,gspd-1(RNAi)n=858. Fordaf-7;idh-1: EVn=1098,gspd-1(RNAi)n=834. Inb,c,d,f, representative images from at least two experiments. Ina,e,g, data were collected from at least five biological replicates, from at least three independent experiments. Error bars represent 95% confidence intervals. Means, confidence intervals and statistical significance were modelled by beta regression analysis. ***P<0.001, **P<0.01, ns no significant difference (beta regression). Figure 3: Cellular NADPH levels determine dauer formation. ( a ) High concentration of trehalose in the feeding medium does not enhance the Daf-c phenotype of daf-7 . Control (water) n =684, trehalose treated n =612. ( b ) 2D-TLC of nucleotides from daf-2(e1370) and daf-2(e1370); ΔΔ tps L3 and dauer larvae. ΔΔ tps causes marked increase in NADPH in both L3 and dauer larvae of daf-2 . ( c ) TLC of sugars from daf-2(e1370) and daf-2(e1370); ΔΔ tps dauers. Note the disappearance of the trehalose band and the accumulation of G6P in daf-2; ΔΔ tps (G6P—glucose-6-phosphate R f ∼ 0.17, Tre—trehalose R f ∼ 0.46, Glu—glucose R f ∼ 0.57). ( d ) 2D-TLC of nucleotides derived from wild-type (N2) L3 larvae after two generations on empty vector control RNAi (EV) or gspd-1 (RNAi) and idh-1(ok2832) on EV. Note the reduction of the NADPH levels caused by gspd-1 (RNAi). The mutant of idh-1 also displays lower NADPH amounts compared with the wild type. Scans of whole TLC plates are shown in Supplementary Figs 3–5 . ( e ) Dauer formation of daf-7 and daf-7; ΔΔ tps on gspd-1 (RNAi) at 20 °C. gspd-1 (RNAi) leads to an increase in the incidence of dauers. For daf-7 : EV n =775, gspd-1 (RNAi) n =782. For daf-7; ΔΔ tps : empty vector n =814, gspd-1 (RNAi) n =734. ( f ) When PPP is partially inactivated by RNAi against gspd-1 , in the first generation the wild-type worms do not have obvious defects. Under the same conditions, idh-1 mutants display pronounced slow growth, sick and reduced body size phenotypes. Scale bars, 500 μm. ( g ) Dauer formation of daf-7 and daf-7;idh-1 on gspd-1 (RNAi) at 20 °C. daf-7;idh-1 shows higher incidence of dauers compared with daf-7 and it is further enhanced by gspd-1 (RNAi). For daf-7 : empty vector n =823, gspd-1 (RNAi) n =858. For daf-7;idh-1 : EV n =1098, gspd-1 (RNAi) n =834. In b , c , d , f , representative images from at least two experiments. In a , e , g , data were collected from at least five biological replicates, from at least three independent experiments. Error bars represent 95% confidence intervals. Means, confidence intervals and statistical significance were modelled by beta regression analysis. *** P <0.001, ** P <0.01, ns no significant difference (beta regression). Full size image As mentioned above, trehalose is synthesized from G6P and UDP-glucose. G6P is an important molecule that stands on the crossroads of several carbohydrate pathways. One such pathway is the PPP. NADPH, a major cellular reducing agent, is essential for a wide array of anabolic processes. NADPH in the cytosol is predominantly produced from G6P in the oxidative phase of the PPP [28] . Thus, trehalose and NADPH biosyntheses are coupled by their common substrate. The electron donor in oxygenation reactions catalysed by microsomal Cyp450 systems is almost exclusively NADPH [29] . DAF-9, as a member of the Cyp450 family, is expected to also use NADPH during DA biosynthesis. Indeed, in vitro reactions with microsomes containing DAF-9 demonstrated a requirement for NADPH [13] . We hypothesized that increased trehalose biosynthesis would reduce the cellular NADPH level by reducing G6P consumption through the PPP. In turn, this would be expected to decrease the DA level and increase dauer formation. Accordingly, reduced TPS activity would be expected to increase the NADPH level by increasing the amount of G6P. To determine the effect of tps-1 / tps-2 on the NADPH level, we designed an extraction procedure to recover nucleotides from worms. Using a 2D-TLC ion-exchange system to visualize NADPH in the nucleotide pool, we compared the NADPH levels in reproductive and dauer larvae. To produce large amounts of worms for biochemical analysis, we made use of the temperature-sensitive Daf-c mutant daf-2(e1370). This mutant produces ∼ 100% L3 larvae at 15 °C and ∼ 100% dauer larvae at 25 °C. Generally, the NADPH levels in both L3 and dauer larvae are very low compared with those of other nucleotides such as ATP/ADP and GTP/GDP ( Fig. 3b and Supplementary Fig. 3 ). This makes NADPH a suitable target for the regulation of Cyp450 activity. Reproductive L3 larvae showed higher levels of NADPH than those of dauer larvae ( Fig. 3b and Supplementary Fig. 3 ). According to our hypothesis, TPS-1/2-deficient worms should produce more NADPH than worms with intact TPS enzymes. Indeed, both L3 and dauer larvae of the daf-2; ΔΔ tps mutant exhibited higher NADPH levels than those of corresponding stages of the daf-2 mutant ( Fig. 3b and Supplementary Fig. 3 ). Moreover, the G6P level was higher in the dauer larvae of daf-2; ΔΔ tps than in those of daf-2 ( Fig. 3c and Supplementary Fig. 4 ). Next, we tested whether the depletion of cytosolic NADPH enhances dauer formation. The first and rate-limiting enzyme of the PPP, G6P dehydrogenase, produces NADPH and phosphogluconolactone from G6P in the cytosol [28] . Inactivation of this enzyme disrupts the entire oxidative phase of the PPP and leads to grave pathologies, such as haemolytic anaemia, due to a decreased redox potential [28] . This enzyme is encoded by a single gene in C. elegans , gspd-1 . Loss-of-function mutations of gspd-1 are lethal; therefore, we decided to use an RNA interference (RNAi) approach. RNAi against gspd-1 had a strong pleiotropic phenotype of slow growth and a sick appearance, but not of constitutive dauer formation, in reproducing wild-type worms of the second generation [30] . The worms also displayed markedly lower NADPH levels ( Fig. 3d and Supplementary Fig. 5 ). Remarkably, two generations of RNAi of gspd-1 in the daf-7 or daf-7; ΔΔ tps backgrounds led to ∼ 100% dauer formation at 20 °C ( Fig. 3e ). Apart from the oxidative phase of the PPP, the second source of cytosolic NADPH in cells is oxidative decarboxylation of isocitrate to 2-oxoglutarate by the enzyme isocitrate dehydrogenase 1 (cytosolic) [31] . In C. elegans , this enzyme is encoded by the gene idh-1 . The mutant idh-1(ok2832) , which bears a large insertion/deletion that eliminates a substantial part of the idh-1 -coding region, is viable, presumably because the PPP continues to furnish a sufficient level of cytosolic NADPH ( Fig. 3d and Supplementary Fig. 5 ). Indeed, when RNAi against gspd-1 was applied to idh-1 , it resulted in a strong growth delay, a sick appearance and a small body size as early as the first generation ( Fig. 3f ). This treatment, however, did not result in a Daf-c phenotype. To test the influence of idh-1 on dauer formation, we produced a daf-7(e1372);idh-1(ok2832) double mutant. At 20 °C, daf-7;idh-1 produced ∼ 26% more dauers than daf-7 ( Fig. 3g ). When PPP was inhibited by gspd-1 (RNAi), the formation of dauers in daf-7;idh-1 in the first generation was increased to >90% ( Fig. 3g ). Therefore, the level of cytosolic NADPH directly regulates dauer formation. DAF-16 and DAF-12 regulate cytosolic NADPH levels As shown above, the biosynthesis of trehalose influences the dauer developmental transition by interfering with the synthesis of NADPH and DA. However, it remained unclear how this process is used in C. elegans as a mechanism to regulate dauer formation. We considered DAF-16 to be one of the possible candidates for regulating this process. It was previously demonstrated that the inhibition of insulin signalling and subsequent activation of DAF-16 leads to the upregulation of tps-1 and tps-2 in the determination of adult longevity and adaptation to hyperosmotic conditions [32] , [33] . In dauer formation, however, one of the main functions of DAF-16 is to regulate the activity of DAF-9 and, consequently, DAF-12 (ref. 34 ). Thus, during dauer formation, DAF-16 might induce the expression of tps-1 / tps-2 via activation of DAF-12 or via an independent mechanism. Conversely, we recently showed that DAF-12 regulates dauer formation via a negative feedback loop by decreasing one of the substrates used for DA synthesis, cholesterol. DAF-12 activates STRM-1, a methylase that renders cholesterol unsuitable for DA synthesis [15] . Thus, DAF-16 and/or DAF-12 could act in a similar way to decrease the level of NADPH, the other substrate for DA synthesis, for example, by activation of TPS-1/2 or downregulation of the activity of PPP and/or IDH-1. We tested the contributions of DAF-16 and DAF-12 to cytosolic NADPH levels using conditions/strains in which either DAF-16 was active but DAF-12 was not, or DAF-12 was active but DAF-16 was not. As mentioned above, class II alleles of daf-2 are not suppressed by daf-12 Daf-d mutations and daf-2;daf-12 double mutants typically arrest as dauer-like larvae due to the activation of DAF-16 (ref. 24 ). Conversely, activation of DAF-12 caused by mutation of daf-9 or substitution of the dietary cholesterol with lophenol also induces the formation of arrested dauer-like larvae in daf-16 loss-of-function mutants [25] , [35] . First, we used qRT–PCR to examine the expression of tps-1 and tps-2 in daf-2(e1370) and daf-2(e1370);daf-12(rh61rh411) worms. Worms were grown at 25 °C to induce arrest as dauer ( daf-2 ) or dauer-like ( daf-2;daf-12 ) larvae. Expression of tps-1 and tps-2 in these worms was compared with that in L3 larvae of the same strains grown at 15 °C. Pronounced upregulation of tps-1 and tps-2 was observed in daf-2 dauers ( Fig. 4a ). In daf-2;daf-12 dauer-like animals, tps-1 and tps-2 were also upregulated, but to a lesser degree than in daf-2 ( Fig. 4a ). Next, we compared the expression of tps-1 and tps-2 in lophenol-induced wild-type (N2) and daf-16(mu86) dauer(-like) larvae with that in cholesterol-grown L3 larvae of the same strains. Both tps genes were upregulated in the dauer(-like) stage, but the upregulation was less pronounced in daf - 16 dauer-like larvae than in N2 dauers ( Fig. 4a ). This demonstrates that DAF-16 and DAF-12 are both sufficient to activate the transcription of tps-1 and tps-2 , but that expression of the tps genes is roughly doubled if both DAF-16 and DAF-12 are active. 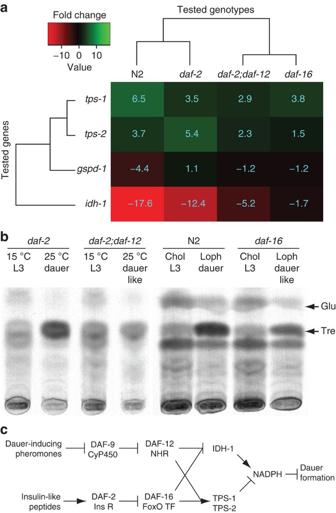Figure 4: DAF-12 and DAF-16 regulate the synthesis of trehalose and NADPH. (a) Heat map of the differential expression ofgspd-1,tps-1,tps-2andidh-1genes indaf-2, daf-2;daf-12, N2 wild-type anddaf-16worms measured using qRT–PCR. The heat map represents the fold change of the expression of the genes in dauer(-like) larvae compared with L3 larvae. (b) TLC of14C-acetic acid-labelled sugars and lipids fromdaf-2anddaf-2;daf-12at 15 or 25 °C and from N2 anddaf-16grown on cholesterol or on lophenol (Tre—trehaloseRf∼0.35; Glu—glucoseRf∼0.5). Scans of whole TLC plates are shown inSupplementary Fig. 6. (c) Dauer formation is controlled by DAF-12 and DAF-16 in a mechanism that involves the production of NADPH. Activation of DAF-12 in response to dauer-inducing pheromones and activation of DAF-16 in response to reduced insulin signalling are both necessary for the activation of TPS-1/2 and the inhibition of IDH-1. As a result, the synthesis of NADPH is diminished and this leads to decrease in DAs and ultimately to dauer formation. Ina, expression levels were measured in three biological replicates. Inb, representative images from two experiments. Figure 4: DAF-12 and DAF-16 regulate the synthesis of trehalose and NADPH. ( a ) Heat map of the differential expression of gspd-1 , tps-1 , tps-2 and idh-1 genes in daf-2, daf-2;daf-12 , N2 wild-type and daf-16 worms measured using qRT–PCR. The heat map represents the fold change of the expression of the genes in dauer(-like) larvae compared with L3 larvae. ( b ) TLC of 14 C-acetic acid-labelled sugars and lipids from daf-2 and daf-2;daf-12 at 15 or 25 °C and from N2 and daf-16 grown on cholesterol or on lophenol (Tre—trehalose R f ∼ 0.35; Glu—glucose R f ∼ 0.5). Scans of whole TLC plates are shown in Supplementary Fig. 6 . ( c ) Dauer formation is controlled by DAF-12 and DAF-16 in a mechanism that involves the production of NADPH. Activation of DAF-12 in response to dauer-inducing pheromones and activation of DAF-16 in response to reduced insulin signalling are both necessary for the activation of TPS-1/2 and the inhibition of IDH-1. As a result, the synthesis of NADPH is diminished and this leads to decrease in DAs and ultimately to dauer formation. In a , expression levels were measured in three biological replicates. In b , representative images from two experiments. Full size image To test whether the decrease in tps-1/2 transcriptional activity in daf-2;daf-12 and daf-16 dauer-like larvae results in decreased synthesis of trehalose, we performed TLC of sugars derived from 14 C-acetate-labelled animals. First, we compared daf-2 and daf-2;daf-12. L3 larvae of both strains contained a basal amount of trehalose, which was higher in daf-2 dauers but unchanged in daf-2;daf-12 dauer-like animals ( Fig. 4b and Supplementary Fig. 6 ). Similarly, 14 C-acetate-labelled N2 lophenol dauers had much higher trehalose levels than those of cholesterol-fed L3 larvae of the same strain. By contrast, the trehalose level in daf-16 lophenol dauer-like larvae was only slightly higher than that in daf-16 L3 larvae ( Fig. 4b and Supplementary Fig. 6 ). Thus, DAF-12 and DAF-16 are both necessary for the increase in trehalose biosynthesis and presumably act at the transcriptional level to modulate the enzymatic activity of TPS-1/2. The abundance of NADPH in the cytosol could also be diminished by downregulation of the activity of PPP NADPH-producing enzymes. However, as shown in Fig. 4a , the expression of gspd-1 in daf-2 and daf-2;daf-12 dauer (-like) larvae is not substantially different from that in L3 larvae. Compared with L3 larvae, gspd-1 ( ∼ 4.4-fold) expression was lower in N2 lophenol dauers; however, almost no change was observed in daf-16 lophenol dauer-like larvae ( Fig. 4a ). Thus, this enzyme does not seem to be regulated at the transcriptional level. As an alternative source of cytosolic NADPH, IDH-1 activity could also be controlled by DAF-16 and/or DAF-12. Indeed, quantitative reverse transcription–PCR (qRT–PCR) analysis showed that idh-1 expression was lower in both daf-2 and daf-2;daf-12 worms at 25 °C than in the same worms at 15 °C ( Fig. 4a ). However, this decrease was much more pronounced in daf-2 ( ∼ 12.4-fold) than in daf-2;daf-12 ( ∼ 5.2-fold). Similarly, N2 lophenol-induced dauers showed a much lower expression level of idh-1 than cholesterol-fed L3 larvae ( ∼ 17.6-fold), whereas idh - 1 expression in daf-16 lophenol-grown dauer-like animals was only ∼ 1.7-fold lower than in daf-16 cholesterol-fed L3 larvae ( Fig. 4a ). These results indicate that DAF-12 and DAF-16 are both necessary for strong downregulation of IDH-1. This finding also suggests that IDH-1, together with TPS-1/2, is a major target of DAF-16 and DAF-12 in the control of cytosolic NADPH levels. This study investigated how carbohydrate metabolism and NADPH availability affect dauer formation. The dauer formation process involves the biosynthesis of trehalose: in mutants unable to synthesize trehalose, dauer formation is strongly reduced. However, our study shows that it is not the presence or absence of trehalose itself that is important for dauer formation, but its biosynthesis. On the basis of our data, we suggest a mechanism to explain how this metabolic pathway regulates dauer formation. TPS-1 and TPS-2 consume G6P in hypodermal cells where DAF-9 is active. G6P is at the crossroads of several carbohydrate pathways, namely, glycolysis, gluconeogenesis, PPP and glycogen and trehalose biosynthesis ( Supplementary Fig. 7 ). G6P is the substrate of the first enzyme of the PPP and is a major source of cytosolic NADPH, a cofactor for DA production. Thus, activation of TPS-1 and TPS-2 results in a decrease in DA synthesis and an increase in dauer formation. Several lines of evidence support the proposed mechanism. First, the use of G6P for trehalose synthesis in worms affects NADPH levels, and these levels correlate with the formation of dauers or entry into the reproductive pathway. Inhibition of GSPD-1 and IDH-1, which are the major enzymes needed for NADPH production in the cytosol, strongly enhances dauer arrest. In addition, RNAi against gspd-1 abolished the effect of the absence of trehalose biosynthesis. Second, the expression patterns of DAF-9 and TPS-1 were very similar. As they are localized to the same cells, regulation via depletion of either substrate or cofactor can be executed within the cell. This is reminiscent of another dauer regulator, STRM-1, which is localized to the hypodermis where methylation of cholesterol occurs [15] . Finally, DAF-16 and DAF-12 inhibited NADPH formation at the transcriptional level by (a) enhancing trehalose biosynthetic enzymes and (b) downregulating IDH-1. In this way, DAF-12, aided by DAF-16, acts in a negative feedback loop that inhibits DA synthesis by decreasing the production of its own ligand. We present the following model based on our observations ( Fig. 4c and Supplementary Fig. 7 ). Dauer-inducing pheromones, through various signalling pathways, act to reduce the activity of DAF-9 (refs 19 , 20 , 34 ). This initial inhibition activates DAF-12, which in turn activates STRM-1 and TPS-1/TPS-2, and inhibits IDH-1. This leads to a decrease in DA caused by the depletion of substrates required for DA production, that is, cholesterol and NADPH. As a result, initial activation of DAF-12 by dauer-inducing pheromones can be enhanced many fold. To be functional, this feedback mechanism requires input from the insulin branch of the dauer-regulatory pathway. The various insulin-like peptides secreted downstream of, but also in parallel to, pheromone-activated pathways converge to regulate the activity of DAF-2 and, consequently, that of DAF-16. The activation of DAF-16 resulting from reduced insulin signalling is necessary for DAF-12-mediated activation of TPS-1/2 and inhibition of IDH-1. Our findings suggest that G6P/NADPH availability regulates the formation of dauers under moderate dauer-inducing conditions. ΔΔ tps does not suppress the Daf-c phenotype of daf-7 at the restrictive temperature, unless the worms are starved in the L1 stage. This observation correlates with the well-known differential regulation of DAF-9 in the hypodermis in response to differences in the strengths of dauer-inducing stimuli [14] , [22] , [36] , [37] , [38] . Under conditions that favour reproductive growth, the XXX cells are the main sources of DAs and DAF-9 is only transiently expressed in the hypodermis. Under such conditions, the liganded DAF-12 activates the expression of genes required for reproductive development, while DAF-16 remains inactive. Trehalose production under such conditions is low and the expression of IDH-1 is high, providing a bigger pool of NADPH for different anabolic processes. However, under moderately dauer-inducing conditions (such as an increase in population density, food shortage and Daf-c mutations at the permissive temperature), DAF-9 activity strongly increases, resulting in the production of enough DA for reproductive development. At this stage, the metabolic activity of the hypodermis determines the outcome of DA production. Enhanced gluconeogenesis and trehalose production in response to the less favourable conditions can gradually deplete the NADPH pool and limit the production of DA. Finally, under strong dauer-inducing conditions, the expression of DAF-9 in the hypodermis is largely shut down so that no DA is produced in this tissue. In this scenario, DAF-12 and DAF-16 activities maintain the low-level production of NADPH, which further limits the production of DA, thereby increasing dauer formation. One of the major conclusions of our study is that a general biochemical pathway can be used as an indicator/executor of a developmental process. The level of G6P that marks the overall metabolic status of the cell determines the amount of a hormone (DA), which in turn determines a developmental transition (reproductive development to dauer formation). Although DA levels are normally regulated by dauer-inducing pheromones or food signals, it now appears probable that the internal metabolic state of the organism also regulates dauer formation. Therefore, we propose a regulatory mechanism that integrates internal metabolic states with dauer signalling pathways to determine dauer developmental fate. Our findings stress the importance of regulating general biochemical processes at the local level in cells. During dauer formation, NADPH, a major reducing agent, is required for the production of fatty acids and depository triglycerides [4] , [39] . A shutdown of the PPP at the organismal level would thus be deleterious for the long-term survival of the dauers. This is why DA and fatty-acid production are spatially separated in the hypodermis and gut, respectively. Lower G6P and NADPH levels in hypodermal cells, induced by the stimulation of trehalose biosynthesis, have no effect on the accumulation of fatty acids and consequently on triglyceride levels in the gut. Future studies may help reveal further interconnections between basic biochemical processes and developmental switches in worms and other organisms. Materials Lophenol was purchased from Research Plus (Manasquan, NJ USA), [1,2,6,7- 3 H]-cholesterol from Biotrends (Cologne, Germany), [1- 14 C]-acetate from HARTMANN ANALYTIC (Braunschweig, Germany), synthetic daumone from KDR Biotech Co. (South Korea) and Dulbecco’s medium from Invitrogen (Karlsruhe, Germany). Short ascaroside derivative of 8 R -hydroxy-2 E -nonenoic acid and (25 S )-Δ 7 -DAs were produced at the Knölker Laboratory [40] , [41] , [42] . All other chemicals were purchased from Sigma-Aldrich (Taufkirchen, Germany). The Caenorhabditis Genetics Centre provided all single mutants. All single mutants were outcrossed at least three times. Compound mutant and transgenic strains were produced during this study or past studies as published [15] , [16] or described below. daf-9(dh6);dhEx24 and daf-9(dh6);daf-12(rh61rh411) were provided by the group of Dr A. Antebi. A list of C. elegans strains can be found in Supplementary Table 1 . Growth and maintenance of worm strains Worms were routinely propagated on nematode growth medium (NGM) agar plates seeded with E. coli NA22 (ref. 43 ). Saturated cultures of E. coli NA22 grown in lysogeny broth (LB) medium were concentrated 10 times and spread on NGM-agar plates. Worms were placed on the plates either as mixed stage populations or as embryos obtained by hypochlorite treatment. The temperature-sensitive Daf-c mutants were grown at 15 °C to grow in the reproductive mode and at 25 °C to arrest as dauer larvae. To obtain lophenol-induced dauer and dauer-like larvae of N2 and daf-16(mu86) , two generations of worms were grown on sterol-depleted solid medium complemented with lophenol [25] . To produce sterol-depleted medium, the agar was replaced by agarose (Sigma-Aldrich) that was washed three times with chloroform to deplete the trace sterols in it. E. coli NA22 was grown in low-glucose, sterol-free DMEM culture medium (Sigma-Aldrich). Bacteria were rinsed with M9 before use. To prepare sterol-containing plates, lophenol or cholesterol 13 mM solutions in ethanol were added to bacteria and the bacteria were spread on the cholesterol-free agarose plates. The final concentration of the sterols was set to 13 μM according to the volume of the agarose plates. Dauer formation assays Overall, 100–150 embryos were transferred to NGM plates seeded with E. coli (NA22), grown at 20 or 25 °C for 3–4 days, and scored for the percentage of dauer larvae. When indicated, trehalose was added to both NGM-agar and bacteria to a final concentration of 200 mM. To determine the effect of starvation during the L1 stage, embryos were transferred to lipid-extracted agarose plates [25] without food and starved for 48 h at 15 °C, and then transferred to NGM plates with E. coli at 25 °C and scored for percentage of dauers. Dauer formation assay with synthetic dauer-inducing pheromones was performed on the basis of previous studies [9] , [15] . Two synthetic dauer-inducing pheromones: daumone (KDR Biotech Co.) and short ascaroside derivative of 8 R -hydroxy-2 E -nonenoic acid [41] were mixed both to NGM and to heat-inactivated NA22 bacteria in equal portions so that the final concentration of each compound was 20 μM. Adult worms were placed to lay eggs ( ∼ 100 eggs per replicate). After 3 days at 25 °C, the plates were scored for dauer formation. To determine dauer formation of daf-9 and daf-9; ΔΔ tps , ∼ 150 bleached embryos of daf-9;dhEx24 and daf-9; ΔΔ tps;dhEx24 were examined on NGM plates with E. coli . Another fraction was starved in L1, as described above, and then transferred to plates with food. dhEx24 is an extrachromosomal array carrying active DAF-9 and nuclear GFP [14] . After 3 days daf-9 and daf-9; ΔΔ tps were identified on the basis of the absence of GFP signal and dauer formation was scored. Formation of the wild type and ΔΔ tps dauers on lophenol-containing plates was examined in the following way [25] . Two generations of worms were grown on sterol-depleted solid medium complemented with lophenol, and dauer formation was determined in the second generation. When indicated, second-generation L1 larvae were starved as described above. In all dauer formation assays, data were collected from at least five biological replicates obtained from at least two experiments. The sample size of each biological replicate was between 45 and 300 animals to ensure power to detect changes in dauer formation. Animals were excluded from the analysis in case of premature embryonic or larval arrest. No randomization was used and the investigator was not blinded during the experiments. A generalized linear model on the basis of beta distribution and logit transformation (beta regression) was used to calculate and compare average dauer formation rates between groups [5] , [44] . The data were tested for meeting the assumptions of the beta distribution, an estimation of the variance was made and groups were statistically compared when the variance between them was similar. Confidence intervals were also estimated from the model and were represented by error bars. RNAi by feeding RNAi against gspd-1 was performed with E. coli HT115 double-stranded RNA (dsRNA)-producing strain from the Ahringer dsRNA-feeding library [30] of Source BioScience (UK). The construct was sequence-verified and shown to contain a large overlap with the coding sequence of gspd-1 ( Supplementary Fig. 8 ). RNAi was performed in two different ways, as indicated in the text. First, for testing the RNAi in the first generation, bleached embryos were seeded to RNAi plates and the resulting worms were grown at 20 °C and scored for phenotypes. Second, for the examination of the effects of RNAi in the second generation, RNAi was induced at the L3/L4 stage of worms grown at 15 °C. Bleached embryos from the resulting adults were seeded to fresh RNAi plates, grown at 20 °C for 3–4 days and scored for phenotypes or used for biochemical analysis. Metabolic labelling Cholesterol labelling . Approximately 3,000 embryos were seeded on NGM plates containing ∼ 10 μCi of [1,2,6,7- 3 H]-cholesterol added to NA22 bacteria and grown for 4 days until early adulthood. At this stage, worms were snap-frozen and stored at −80 °C. Acetic acid labelling . Approximately 20,000 synchronized L1 larvae were put on seeded plates containing 10–20 μCi of [1- 14 C]-acetic acid and grown for 3–4 days at 15 or 25 °C until L3 reproductive larvae or dauer/arrested larvae were formed, respectively. Worms were snap-frozen and stored at −80 °C. Lipid and sugar extraction and TLC analysis For metabolic labelling, worms were grown as described above. For non-radioactive lipid analysis, ∼ 20,000 synchronized L1 larvae were seeded on NGM plates with NA22 bacteria and grown at 25 °C for 3 days to form dauer larvae. Worms were lysed by freezing/thawing and extracted by using the Bligh and Dyer method [45] . After phase separation, lipids and sugars were recovered from the lower and upper phases, respectively. After drying and concentration, the non-radioactive samples were normalized for the protein content of the lysate. Radioactive cholesterol and acetic acid-labelled samples were normalized for total radioactivity. Acidic compounds in 3 H-cholesterol samples were enriched on QAE diethyl-(2-hydroxy-propyl)aminoethyl (QAE) Sephadex (40–125 μm beads) ion-exchange column (Sigma-Aldrich). To equilibrate the column, 0.2 g of QAE Sephadex were incubated in 10 volumes of 0.2 N HCl for 30 min, washed with water to pH 7, incubated with 10 volumes of 0.2 N NaOH for 30 min, washed again with water to pH 7 and incubated in 10 volumes of 0.1 N acetic acid. Finally, the column was washed with 10 volumes of methanol, the samples were applied, washed with 10 ml of methanol and eluted with 10 ml of 0.2 N acetic acid dissolved in methanol. Samples were dried, concentrated and applied to TLC plates. TLC was performed on 10-cm HPTLC plates (Merck, Darmstadt, Germany). Sugars were separated using chloroform–methanol–water (4:4:1) or butanol–ethanol–water (5:3:2, two consecutive TLC runs) as the running system. 2D-TLC for the detection of DAs was conducted using chloroform–methanol (24:1) as first system and chloroform–methanol–32% ammonia (60:35:5) as the second system [15] . TLC plates were sprayed with Molisch reagent for sugar detection. TLC plates containing radioactive samples were sprayed with scintillation fluid (Lumasafe, Lumac LSC B.V., Groningen, the Netherlands) and exposed to X-ray film (Kodak Biomax MR, Sigma-Aldrich). Extraction and TLC analysis of NADPH Worms ( ∼ 30,000 dauer or L3 larvae) were grown as described above, collected and washed in ddH 2 O, and pelleted by centrifugation. The worm pellets were snap-frozen in liquid nitrogen and stored at −80 °C. To the frozen worm pellets 0.71 ml of cold methanol was added, followed by sonication in ice-cold sonication bath for 10 min. The resulting methanol homogenates were vigorously mixed and left on ice for 30 min. Methyl tert -butyl ether (2.135 ml) was added and the sonication followed by mixing and incubation on ice was repeated. ddH 2 O (0.985 ml) was added and, after sonication and vigorous mixing, the samples were left on ice for 1 h. The suspensions were centrifuged at 4,500 r.p.m. for 10–20 min to facilitate the phase separation. The lower (aqueous) phases were collected and concentrated via drying in a speed-vac concentrator until the volume of the samples reached 200 μl. The volume of the samples was corrected with ddH 2 O according to previously measured protein content and 100 μl of them were applied to polyethylenimine (PEI)-cellulose 20 × 20 cm TLC plates (Merck). 2D-TLC was performed following a procedure modified from a previous study [46] . The first dimension was performed as a stepwise elution with 0.2 M LiCl (2 min), 1 M LiCl (6 min) and 1.6 M LiCl (to the end) without drying of the TLC plates in between. After the first dimension was completed, the wet TLC plates were immersed in 100% methanol for 20 min and dried under nitrogen flow. The second dimension was performed as a stepwise elution with sodium formate—formic acid buffers, pH 3.4 in the following order: 0.5 M buffer (30 s), 2 M buffer (2 min) and 4 M buffer (to the end). After drying the plates under nitrogen flow, the TLC plates were examined under ultraviolet source (254 nm). Quantitative real-time PCR The differential expression of gspd-1 , tps-1 , tps-2 and idh-1 genes was measured using qRT–PCR. daf-2(e1370) and daf-2(e1370);daf-12 were grown at 15 °C or 25 °C to obtain L3 larvae or dauer/dauer-like larvae, respectively. N2 and daf-16(mu86) were grown on cholesterol or lophenol-containing plates to obtain L3 larvae or dauer/dauer-like larvae, respectively [25] . Total RNA was isolated using the PureLink RNA Mini Kit (Ambion) and equal amounts of all samples were reverse transcribed with SuperScript III (Invitrogen) using oligo(dT) 12–18 primers. cDNA quality was tested using standard PCR. qRT–PCR was performed on Stratagene Mx3000P (Agilent Technologies) with at least three samples in duplicates. Primer sequences are presented in Supplementary Table 2 . Raw SYBR green fluorescence data were analysed in R using the qpcR package version 1.4 (ref. 47 ). A seven-parameter sigmoidal model was fit on each PCR curve. The same model was also used for background subtraction. The second derivative maximum of the fit was defined as the C p value. The efficiency of a PCR reaction was estimated as the mean of all sigmoidal efficiencies in its replicates. Expression levels were averaged over technical and biological replicates, and normalized to the expression level of the mrlp-40 gene via permutation approach. Generation of daf-9 ;ΔΔ tps tps-1 males were crossed to daf-9(dh6);dhEx24 and then GFP-positive hermaphrodites from the first generation were crossed to tps-1 males. Self-fertilization of second-generation GFP-positive hermaphrodites gave third generation of GFP-positive hermaphrodites and these worms were singled to give daf-9(dh6),tps-1(ok373);dhEx24 . The strains were selected for being GFP-positive, homozygous for tps-1 (tested using PCR), and producing dauer-like larvae. daf-9(dh6),tps-1(ok373);dhEx24 hermaphrodites were then crossed to tps-2 males, and GFP-positive males from the progeny were backcrossed to daf-9(dh6),tps-1(ok373);dhEx24 . Second-generation GFP-positive hermaphrodites were self-fertilized to give fraction of tps-2(ok526);daf-9(dh6),tps-1(ok373);dhEx24 worms in the third generation. Strains were again controlled for GFP signal; PCR for verification of the homozygous state of tps-2 and tps-1 was carried out and the Daf-c phenotype was inspected. Generally, none of the tps-2(ok526);daf-9(dh6),tps-1(ok373);dhEx24 strains were able to produce GFP-negative L4 larvae or adult worms. For the production of such worms, (25S)-Δ 7 DA was added to the feeding media, which resulted in the formation of fertile adult daf-9(dh6); ΔΔ tps . Generation of daf-2(e1368); ΔΔ tps daf-2(e1368) males were crossed to tps-2(ok526);tps-1(ok373) hermaphrodites and the resulting males were backcrossed to tps-2(ok526);tps-1(ok373) . The second-generation hermaphrodites were separated to self-fertilize. Third-generation larvae were grown on non-permissive temperature (25 °C) and individuals, which developed into dauer larvae, were selected. These were shifted to permissive temperature (15 °C) so that they could exit from the dauer state and self-fertilize to give fraction of triple-homozygous tps-2(ok526);daf-2(e1368);tps-1(ok373) mutants. Strains were quality-controlled using PCR and dauer phenotypic assays. Generation of daf-7;idh-1 Males heterozygous for idh-1(ok2832) were crossed to daf-7(e1372) hermaphrodites. The hermaphrodites from the progeny laid eggs that at 25 °C developed into dauers or adults. The dauers were relocated to 15 °C to re-enter reproduction and their progeny was screened using PCR for homozygous daf-7(e1372);idh-1(ok2832) individuals. Overexpression of tps-1 ::eGFP in daf-7 The tps-1 -containing fosmid WRM0628cF08 was recombineered by C-terminal tagging of the tps-1 gene (ZK54.2) with eGFP optimized for C. elegans . This was performed via a procedure modified from literature [48] where improved plasmids pRedFlp4 and pPUBH were used instead of the original pRedFlp and pPUB. However, WRM0628cF08 contained several additional genes. To eliminate them, the construct was engineered so that only eGFP-tagged tps-1 -coding sequence with its corresponding 5′- and 3′-untranslated repeats and ∼ 5 kB promoter region remained in it ( Fig. 2a ). For that, a subcloning cassette was prepared using PCR amplification from the pPUBH plasmid using a specific pair of primers. The sequences of the primers can be seen in Supplementary Table 3 . The first 50 bp (homology arms) are specific to the tps-1 sequence; the rest of the sequence is specific to pPUBH plasmid sequence. The host cells containing the original fosmid construct were transformed with the subcloning cassette via electroporation. Transformants were selected by blasticidin resistance and the presence of the new construct was confirmed via fingerprinting by XbaI digestion. The new construct was then bombarded into unc-119 worms and eGFP-positive worms without unc phenotype were selected. The progeny of these transgenes was followed for several generations and, according to the segregation of the eGFP signal, it was confirmed that the construct existed as an extrachromosomal array. To introduce the tps-1 ::eGFP in daf-7(e1372) background, tps-1 ::eGFP was first outcrossed twice to N2 and then eGFP-positive males were crossed to daf-7 hermaphrodites. eGFP-positive hermaphrodites of the progeny were let to lay eggs at 25 °C to form eGFP-positive dauer larvae, which would be candidates for homozygous daf-7 with tps-1 ::eGFP. eGFP-positive dauer larvae were singled in 12-well NGM plates with NA22 bacteria and supplemented with 1.3 μM (25S)-Δ 7 DA to resume reproductive development. Strains were examined for several generations for dauer formation and strong eGFP signal. How to cite this article: Penkov, S. et al. Integration of carbohydrate metabolism and redox state controls dauer larva formation in Caenorhabditis elegans . Nat. Commun. 6:8060 doi: 10.1038/ncomms9060 (2015).